A single site ruthenium catalyst for robust soot oxidation without platinum or palladium The quest for efficient non-Pt/Pd catalysts has proved to be a formidable challenge for auto-exhaust purification. Herein, we present an approach to construct a robust catalyst by embedding single-atom Ru sites onto the surface of CeO 2 through a gas bubbling-assisted membrane deposition method. The formed single-atom Ru sites, which occupy surface lattice sites of CeO 2 , can improve activation efficiency for NO and O 2 . Remarkably, the Ru 1 /CeO 2 catalyst exhibits exceptional catalytic performance and stability during auto-exhaust carbon particle oxidation (soot), rivaling commercial Pt-based catalysts. The turnover frequency (0.218 h −1 ) is a nine-fold increase relative to the Ru nanoparticle catalyst. We further show that the strong interfacial charge transfer within the atomically dispersed Ru active site greatly enhances the rate-determining step of NO oxidation, resulting in a substantial reduction of the apparent activation energy during soot oxidation. The single-atom Ru catalyst represents a step toward reducing dependence on Pt/Pd-based catalysts. Auto-exhaust carbon particles (mainly containing soot) constitute a major source of atmospheric pollution, leading to severe environmental and health problems [1] , [2] . To address this problem effectively, a catalytic after-treatment technique combining particulate filters and oxidation catalyst has been adopted as the most effective strategy [3] , [4] . The success of this approach heavily relies on high-efficiency catalysts that facilitate soot oxidation at lower temperature range [5] . Researchers have explored numerous high-efficient catalysts for soot oxidation, including precious metal and metal oxides [6] , [7] , [8] . Notably, platinum (Pt) and palladium (Pd) metals remain essentially active components in commercial catalysts for soot purification, with their usage exceeding 42 % of the global demand amount, as reported in the Pgm market report (May 2023) by Johnson Matthey. This high reliance on Pt/Pd significantly contributes to the costly nature of auto-exhaust after-treatment systems. Developing high-efficiency, non-Pt/Pd catalysts with lower costs for soot oxidation presents a challenging task [9] . While the cost of ruthenium (Ru) metal is merely a third of Pt/Pd, the creation of Ru-based catalysts exhibiting both high activity and stability has been rarely reported in vehicle catalysts [10] , [11] . The primary issue lies in the volatility of Ru oxides at higher temperatures [12] , [13] . Hence, designing and preparing a robust and cost-effective Ru-based catalyst for auto-exhaust applications, capable of inhibiting volatile Ru at elevated temperatures, holds great significance in replacing Pt/Pd-based catalysts in the field of soot purification. Studies have found that the strong interactions between Ru and CeO 2 in the Ru/CeO 2 catalyst can enhance the catalytic activity and the thermal stability during soot oxidation reaction [14] . Therefore, employing a strong metal-support interaction (SMSI) emerges as a reasonable strategy to enhance the stability of Ru-based catalysts. Nonetheless, fabricating high-efficiency Ru-based catalysts with optimal atomic configurations continues to present a formidable challenge. In recent times, single-atom catalysts (SACs) have garnered significant attention, especially precious metal SACs, due to their exceptional atomic utilization and uniform active site structure, making them highly attractive for deep oxidation reactions [15] , [16] . Studies further reveal that the architecture interfacial sites in SACs catalysts significantly influence both catalytic performance and thermal stability [17] , [18] , [19] , [20] . The complexity of soot oxidation occurring at the three-phase interface among solid catalysts, soot particles, and gaseous reaction gases (O 2 and NO), adds to the challenge of designing and preparing efficient SACs catalysts [21] . This complexity demands careful consideration of both the intrinsic activity and stability of the catalyst for adsorbed/activated reactants, and the contact efficiency between soot particles and catalysts, as these factors play crucial roles in the reaction [22] , [23] , [24] , [25] , [26] , [27] . Compared to other oxides, Ceria (CeO 2 ) proves to be an excellent cocatalyst, enhancing the catalytic performance and stability of precious metal active components in auto-exhaust catalysts because of its excellent oxygen storage/release properties [28] , [29] , [30] . In our previous works, we successfully constructed a series of Ce-based oxides as supports for the preparation of highly efficient supported noble metal soot oxidation catalysts [31] . Furthermore, our works highlight the importance of the strong interaction between Au NPs and CeO 2 with the optimal crystal facet, which is crucial to adjust the intrinsic activity for O 2 activation [32] . Despite these advancements, there remains limited research on SACs of single-atomic Ru anchored at the surface lattice of single-crystal CeO 2 , which holds the potential for replacing Pt/Pd-based catalysts in the field of soot purification. In this study, we present a simple one-step synthesis of stabilized single-atom Ru sites confined on the surface lattice site of nanoflower-like CeO 2 microspheres (Ru 1 /CeO 2 ) using the gas bubbling-assisted membrane deposition (GBMD) method. These single-atom Ru active sites demonstrate remarkable thermal stability and enhance the activation efficiency of reactants (NO and O 2 ). The Ru 1 /CeO 2 catalyst, with Ru single sites on the CeO 2 surface, exhibits excellent intrinsic catalytic performance and stability during soot oxidation under a loose contact model, outperforming both Ru nanoparticle and commercial Pt-based catalysts. Through comprehensive characterizations and density functional theory calculations, we identify the atomically dispersed Ru 1 O 5 active site in the Ru 1 /CeO 2 catalyst, along with the strong interface charge transfer within the Ru-O-Ce bond. The well-constructed active sites facilitate the formation of crucial surface NO 2 * intermediate species, which play a key role in the rate-determining step of NO oxidation to NO 2 , resulting in a significant reduction of the apparent activation energy during catalytic soot oxidation. This work emphasizes the advantages of synthesizing well-defined catalytic single sites on nanocrystals, and the combination of in-situ DRIFTS and DFT calculations provides valuable insights into the reaction mechanism. Furthermore, it establishes a methodological foundation for obtaining high-efficiency catalysts for auto-exhaust purification. The single-atom Ru catalyst offers a highly promising and cost-effective solution for auto-exhaust treatment systems. Chemical structure characterizations of Ru 1 /CeO 2 and Ru n /CeO 2 catalysts The detailed synthesized processes of nanoflower-like CeO 2 microspheres and Ru 1 /CeO 2 catalyst were described (Supplementary Fig. 1 ) . The atomically dispersed Ru 1 /CeO 2 catalyst was synthesized using the GBMD method [33] , while the reference catalyst of supported Ru nanoparticles (NPs) on nanoflower-like CeO 2 (Ru n /CeO 2 ) was obtained through the gas bubbling-assisted membrane reduction method [34] . 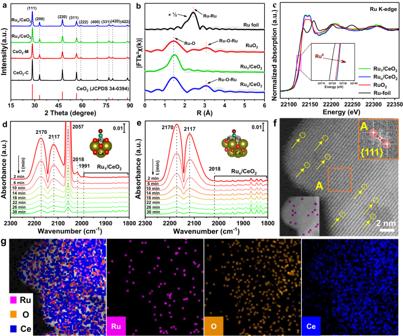Fig. 1: Structure characterization of Ru1/CeO2and Run/CeO2catalysts. aXRD patterns of all samples and standard card of CeO2.bEXAFS fitting results in R space and the Ru K- edge for Ru1/CeO2and Run/CeO2catalysts with RuO2and Ru foil. The shell radii (R) of Ru-O and Ru-O-Ru are marked.cThe Ru K-edge XANES profiles.dandeIn-situ DRIFT spectra of CO adsorption at 50oC for the Ru1/CeO2and Run/CeO2catalysts with the extension of purge time (N2flow, 30 mL min-1).fSTEM-ADF image of Ru1/CeO2catalyst with scale bars of 2 nm. The yellow circles represent atomically dispersed Ru sites.gSTEM EDX mapping of Ru1/CeO2catalyst (Purple, Ru; Orange, O; Mazarine, Ce). Inductively coupled plasma optical emission spectroscopy (ICP-OES) analysis revealed that the actual Ru loading amounts in Ru 1 /CeO 2 and Ru n /CeO 2 catalysts are 0.46 wt.% and 3.80 wt.%, respectively (Supplementary Table 1 ). The powder X-ray diffraction (XRD) patterns of all samples exhibit characteristic peaks of CeO 2 nanocrystals with a cubic fluorite structure (JCPDS 34-0394). Notably, no characteristic diffraction peaks associated with Ru or RuO x NPs are detected, implying that the Ru species are highly dispersed on the surface of CeO 2 (Fig. 1a ). The lattice constant of CeO 2 in the Ru 1 /CeO 2 catalyst slightly decreases to 5.4084 Å compared to pure CeO 2 (5.4101 Å) (Supplementary Table 1 ). This decrease is attributed to the substitution of Ce-sites on the surface lattice by smaller cation radius Ru ions (Supplementary Fig. 2 ). The SEM and TEM images provide a detailed view of the monodispersed nanoflower-like CeO 2 microspheres, composed of single-crystal nanosheets (Supplementary Figs. 3a– d and 4 ). The thickness of these nanosheets is about 18 nm (Supplementary Fig. 5a, b ), and the distance between two Ce atoms measures 3.1 Å, with clear step sites observed at the edge of the nanosheets (Supplementary Fig. 6 ). Fig. 1: Structure characterization of Ru 1 /CeO 2 and Ru n /CeO 2 catalysts. a XRD patterns of all samples and standard card of CeO 2 . b EXAFS fitting results in R space and the Ru K- edge for Ru 1 /CeO 2 and Ru n /CeO 2 catalysts with RuO 2 and Ru foil. The shell radii ( R ) of Ru-O and Ru-O-Ru are marked. c The Ru K-edge XANES profiles. d and e In-situ DRIFT spectra of CO adsorption at 50 o C for the Ru 1 /CeO 2 and Ru n /CeO 2 catalysts with the extension of purge time (N 2 flow, 30 mL min -1 ). f STEM-ADF image of Ru 1 /CeO 2 catalyst with scale bars of 2 nm. The yellow circles represent atomically dispersed Ru sites. g STEM EDX mapping of Ru 1 /CeO 2 catalyst (Purple, Ru; Orange, O; Mazarine, Ce). Full size image In the N 2 adsorption-desorption isotherms, all catalysts exhibit an H4 hysteresis loop in the P/P 0 range 0.4-1.0, indicating the presence of a porous structure in the as-prepared samples (Supplementary Fig. 7a ). The pore size distribution profiles of nanoflower-like CeO 2 , Ru 1 /CeO 2 , and Ru n /CeO 2 catalysts all exhibit two peaks centered at 4.5 and 13.0 nm, in contrast to the single peak observed for CeO 2 -C at 8.0 nm (Supplementary Fig. 7b ). The formation of these pores is attributed to the interwoven CeO 2 nanosheets and stacked CeO 2 nanoparticles (Supplementary Fig. 8a, b ). To investigate the local electronic structure and coordination environment of Ru in the Ru/CeO 2 catalysts, X-ray absorption measurements were conducted. The extended X-ray absorption fine structure (EXAFS) of Ru 1 /CeO 2 shows only a primary peak at 1.49 Å, while the Ru n /CeO 2 catalyst exhibits two peaks at 1.49 and 3.07 Å (Fig. 1b ), corresponding to the Ru-O and Ru-O-Ru bond, respectively [35] , [36] . Further EXAFS curves fitting analyses provide insights into the coordination environment of Ru species in Ru 1 /CeO 2 and Ru n /CeO 2 catalysts, giving the coordination number of nearest-neighbor O atoms surrounding the isolated Ru atom (Fig. 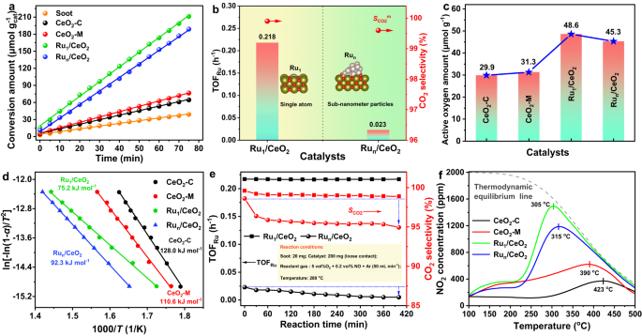Fig. 2: Catalytic performances of Ru1/CeO2and Run/CeO2catalysts in soot oxidation. aSoot conversion amount as a function of times by isothermal oxidation reaction at 280oC.bTOFRuover Ru1/CeO2and Run/CeO2catalysts.cActive oxygen amount by isothermal anaerobic titration at 280oC.dOzawa plots of ln[-ln(1-α)/T2] vsT-1for different soot conversion.eTime-TOFRuand the selectivity of CO2over Ru1/CeO2and Run/CeO2catalysts (Reaction condition: Soot, 20 mg; Catalyst, 200 mg; Reactant gas flow, 50 mL min-1; At 280oC).fNO2concentration curves of NO temperature-programmed oxidation. 1b and Supplementary Table 2 ). The coordination number of O atoms surrounding Ru atom in Ru 1 /CeO 2 catalyst is 5.3, with a mean bond length of 2.01 Å, while the value of Ru n /CeO 2 catalyst is 3.4, with the bond length of 2.04 Å. As a result, the atomically dispersed Ru species in the Ru 1 /CeO 2 catalyst diffuse into the surface lattice of CeO 2 , forming coordination unsaturated Ru 1 O 5 active sites. The atomic dispersion of Ru species in the Ru 1 /CeO 2 catalyst is further corroborated by subsequent characterizations. The X-ray photoelectron spectroscopy (XPS) spectra of Ru 1 /CeO 2 and Ru n /CeO 2 catalysts were acquired to determine the status of Ru species. The Ru 3 p spin-orbit splits into 3 p 3/2 and 3 p 1/2 components, corresponding to the binding energy (BE) of 462.2 and 484.1 eV [37] , [38] . The two BE pairs (461.7 and 484.7 eV; 463.3 and 485.3 eV) corresponding to Ru 3 p 3/2 and 3 p 1/2 can be assigned to Ru 0 and Ru n+ species, respectively (Supplementary Fig. 9 ) [39] , [40] . In the Ru 1 /CeO 2 catalyst, the Ru 3 p XPS only shows the oxidation state, indicating the presence of single positively charged Ru atoms. Conversely, the Ru 3 p peak of the Ru n /CeO 2 catalyst exhibits the coexistence of Ru 0 and Ru n+ (4 ≤ n ≤ 6) species, attributed to the formation of a core-shell structured Ru@RuO x layer in Ru sub-nanometric particles (SNPs) [41] . This suggests that the Ru species in the Ru 1 /CeO 2 catalyst consist of single-atom Ru with a positively charged feature, while the Ru species in Ru n /CeO 2 catalyst contain a certain amount of metallic state. Furthermore, the Ru K-edge adsorption position of the near-edge X-ray absorption fine structure (NEXAFS) spectra over the Ru 1 /CeO 2 catalyst is slightly higher than that of Ru n /CeO 2 and RuO 2 observed through local magnification (Fig. 1c ). This observation indicates that the valence state of single-atom Ru species in the Ru 1 /CeO 2 catalyst is higher than +4, consistent with the result obtained from the Ru 3 p XPS analysis. Diffuse reflectance infrared Fourier transform spectrum of CO adsorption (CO-DRIFTS) on noble metal catalysts is widely used to investigate the atomic and electronic structures of metal-support binding sites. In the case of Ru/CeO 2 catalysts, CO-DRIFTS can differentiate between active Ru sites in single atoms and nanoparticles. The CO-DRIFTS spectrum of Ru 1 /CeO 2 catalyst shows four strong adsorption peaks (Fig. 1d ), whereas the spectrum of Ru n /CeO 2 catalyst shows only two strong adsorption peaks (Fig. 1e ). The strong adsorption peaks centered at 2170 and 2117 cm -1 are assigned to the R and P branches of the rotation vibrational spectra of gas-phase CO species [42] . The strongest peak centered at 2057 cm -1 is ascribed to the C-O stretching vibration of dicarbonyl CO species (Ru n+ (CO) 2 ) adsorption on single atomically dispersed Ru n+ sites [43] , [44] , [45] . The peak centered at ~2018 cm -1 can be assigned to C-O vibration of CO linearly bound Ru sites with high coordination [46] , while the peak at ~1991 cm- 1 could be ascribed to the CO adsorbed on oxygen vacancies or Ru-doped CeO 2 [47] . These findings indicate that the Ru species in Ru 1 /CeO 2 catalyst exist as a single atomically dispersed ionic state, forming a Ru-O-Ce bond originating from the surface lattice site of CeO 2 , which has been substituted by a single Ru atom. On the other hand, the CO adsorption peak of the Ru n /CeO 2 catalyst, centered at 2057 cm -1 , is difficult to detect, but it demonstrates two weak bands at 1830 and 1860 cm −1 , which can be attributed to the bridged adsorption of CO on two and three Ru atoms [46] , [48] , indicating the presence of Ru sub-nanometric particles (SNPs). With increasing purging time, the intensity of CO adsorption band on single atomic Ru sites decreases significantly, whereas that on Ru SNPs remains relatively unchanged. This suggests that the binding strength of CO to Ru 1 is lower than that of Ru SNPs. To further visualize the existence and dispersion state of the Ru species, aberration-corrected STEM images of the catalysts were obtained. Upon the introduction of the Ru species, Ru 1 /CeO 2 catalyst maintains the initial nanoflower-like morphology of CeO 2 (Supplementary Fig. 10a, b ). The atomically dispersed Ru species in Ru 1 /CeO 2 catalyst are faintly observed and coincided with the atomic lattice of CeO 2 (Fig. 1f ). The interplanar crystal spacing of CeO 2 paralleled to the edge is 3.1 Å, as determined from the fast Fourier transform (FFT) pattern in the inset (A) of Fig. 1f , and corresponds to the exposed CeO 2 (111) crystal facets. STEM images and corresponding Energy-dispersive X-ray (EDX) element mapping of the Ru 1 /CeO 2 catalyst demonstrate the homogeneous dispersion of single-atom Ru species on the surface of CeO 2 support (Fig. 1g ). In contrast, the Ru species in Ru n /CeO 2 catalyst exhibit a certain degree of aggregation and form small Ru SNPs (Supplementary Fig. 11a, b ). The size distribution and EDX element mapping analysis in STEM-ADF images show the uniformed dispersion of Ru SNPs ( d = 0.9 ± 0.2 nm) deposited on the surface of CeO 2 nanosheets (Supplementary Fig. 12 ). Based on the results of EXAFS, in-situ CO-DRIFTS and STEM characterizations, it is evident that the state of Ru species in Ru 1 /CeO 2 catalyst is predominantly isolated single-atom dispersion, occupying the surface lattice sites of CeO 2 nanocrystals to form Ru 1 O 5 structure. Conversely, the state of Ru species in the Ru n /CeO 2 catalyst is RuO 2 SNPs. Catalytic performance and kinetics of Ru/CeO 2 catalysts in soot oxidation The performance of all catalysts for soot oxidation was evaluated under the loose contact mode. To highlight the catalytic performance of the CeO 2 -M nanosheet catalyst, conventional powder-type CeO 2 (CeO 2 -C) was synthesized as the reference sample. The relative reaction rates ( R ) of catalyzing soot oxidation were calculated through an isothermal oxidation reaction at 280 o C (Fig. 2a ) . The CeO 2 -M catalyst exhibits a higher R value (0.94 μmol g −1 min −1 ) compared to the CeO 2 -C sample (0.79 μmol g −1 min −1 ), indicating that the nanoflower-like morphology effectively enhances catalytic performance for soot oxidation. Additionally, the tight soot-catalyst contact mode over the same catalyst showed higher performance compared with the loose contact mode, which approximates real conditions (Supplementary Fig. 13a, b ). Upon the introduction of Ru species, the R values of Ru 1 /CeO 2 and Ru n /CeO 2 catalysts remarkably increased to 2.59 and 2.38 μmol g -1 min -1 , respectively. The actual Ru content obtained by ICP-OES allowed the representation of the reaction rate per each Ru atom, represented as the turnover frequency (TOF Ru ). The TOF Ru value of Ru 1 /CeO 2 catalyst (0.218 h -1 ) is approximately nine-fold higher than that of Ru n /CeO 2 catalyst (0.023 h -1 ) (Fig. 2b ). This suggests that a single atomic Ru site possesses both high activity and atom utilization. Moreover, the selectivity of CO 2 product ( S CO2 ) over the Ru 1 /CeO 2 catalyst is close to 100 %, allowing for the rapid removal of CO product emitted from vehicle exhaust. 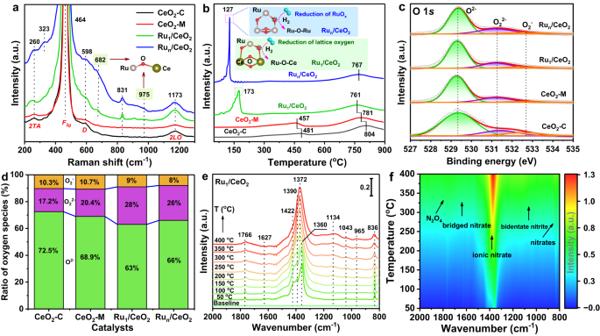Fig. 3: Identifying active species and reaction pathways of the catalysts during catalyzing soot oxidation. aRaman spectrum with an excitation wavelength of 532 nm.bH2-TPR profiles.cXPS spectra of O 1s.dThe ratio of oxygen species determined by XPS.eTemperature-dependent in-situ DRIFT spectra and (f) corresponding contour projection results of NO oxidation on Ru1/CeO2catalyst (Catalyst, 10 mg; 5 vol% O2and 0.2 vol% NO). Furthermore, the Ru 1 /CeO 2 catalyst exhibits excellent intrinsic catalytic performance during auto-exhaust soot oxidation compared to the commercial Pt-based catalysts (Supplementary Table 3 ). Fig. 2: Catalytic performances of Ru 1 /CeO 2 and Ru n /CeO 2 catalysts in soot oxidation. a Soot conversion amount as a function of times by isothermal oxidation reaction at 280 o C. b TOF Ru over Ru 1 /CeO 2 and Ru n /CeO 2 catalysts. c Active oxygen amount by isothermal anaerobic titration at 280 o C. d Ozawa plots of ln[-ln(1- α )/ T 2 ] vs T -1 for different soot conversion. e Time-TOF Ru and the selectivity of CO 2 over Ru 1 /CeO 2 and Ru n /CeO 2 catalysts (Reaction condition: Soot, 20 mg; Catalyst, 200 mg; Reactant gas flow, 50 mL min -1 ; At 280 o C). f NO 2 concentration curves of NO temperature-programmed oxidation. Full size image The amount of active surface oxygen species plays a crucial role in catalytic performance for deep oxidation reactions, and it was determined by isothermal anaerobic titration at 280 o C (Supplementary Fig. 14a-d ). The presence of single atomic Ru species in the Ru 1 /CeO 2 catalyst significantly increased the active oxygen amounts from 31.3 (CeO 2 -M) to 48.6 μmol g -1 (Ru 1 /CeO 2 ), owing to the contribution of interface oxygen species in Ru-O-Ce bond (Fig. 2c and Supplementary Fig. 14a-d ). To explore the reaction energy barrier on single atomic Ru sites during soot oxidation, the Arrhenius plots of the catalysts were analyzed (Fig. 2d ). 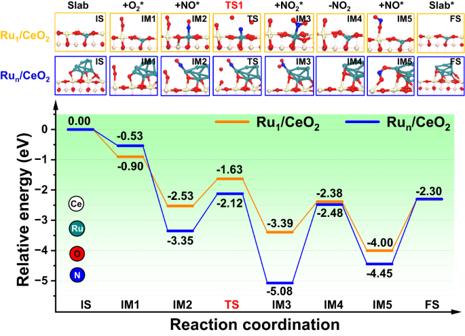Fig. 4: DFT calculations of Ru1/CeO2and Ru10/CeO2catalysts for NO oxidation. Reaction steps during catalyzing NO oxidation (Ru atom, black green; Ce atom, gray; O atom, red; N atom, blue). Color code: Ru1/CeO2(brown line) and Ru10/CeO2(blue line). The Ru 1 /CeO 2 catalyst exhibited the lowest apparent activation energy ( E a , 75.2 kJ mol −1 ) in comparison with CeO 2 and Ru n /CeO 2 catalysts (Supplementary Table 4 ), indicating that single atomic Ru sites play a pivotal role in boosting the catalyzing soot oxidation. Addressing the stability concerns associated with single-atom catalysts, we further investigated the stability of Ru species in the catalysts via the TOF Ru and S CO2 values versus time (Fig. 2e ). The TOF Ru and S CO2 values of the Ru 1 /CeO 2 catalyst remain relatively stable during 400 min, whereas those of the Ru n /CeO 2 catalyst gradually decrease. In line with the cyclic test results of soot oxidation (Supplementary Figs. 15 and 16a, b ), this confirms that the Ru 1 /CeO 2 catalyst demonstrates higher catalytic stability compared with the Ru n /CeO 2 catalyst. Additionally, the morphology and crystal phase structure remain unchanged during six-cycle TPO tests (Supplementary Fig. 17 ). On the other hand, ICP-OES analysis revealed a significant loss of Ru content on the used Ru n /CeO 2 catalyst, which could be attributed to the volatilization of Ru species (Supplementary Fig. 18 ). The Ru 1 /CeO 2 catalyst, with the surface lattice confinement single atom Ru, effectively inhibited the volatilization of Ru species. The CO-DRIFTS of the used Ru 1 /CeO 2 catalyst demonstrated Ru species maintain a single atomically dispersed ionic state (Supplementary Fig. 19a, b ), and STEM EDX mapping of Ru 1 /CeO 2 catalyst also showed high dispersion of Ru species (Supplementary Fig. 20a, b ). Conversely, the Ru species in the Ru n /CeO 2 catalyst had aggregated into larger particles (Supplementary Fig. 21 ). The Ru 3 p XPS spectra of the used Ru 1 /CeO 2 catalyst still maintained the oxidation state with peaks located at 463.3 and 485.3 eV, corresponding to Ru n+ species (Supplementary Fig. 22 ). Raman spectra of the used Ru 1 /CeO 2 revealed that the lattice-confined single-atom Ru 1 /CeO 2 structure remains stable (Supplementary Fig. 23a, b ). However, for the used Ru n /CeO 2 catalyst, the peak intensity of RuO 2 species (~323 cm −1 ) increased, indicating the aggregation of RuO 2 into larger particles after six cycles of soot-TPO tests. After six cycles of tests, the I D /I F2g value (area ratio of D peak to F 2g peak for Raman spectra) of the Ru n /CeO 2 catalyst significantly decreased. This suggests that the interaction between the Ru species and CeO 2 has changed, resulting in a decrease in the number of oxygen vacancies on the CeO 2 surface. Additionally, the surface plasmon resonance (SPR) peak of UV-Vis red-shifted for the used Ru n /CeO 2 catalyst (Supplementary Fig. 24 ), further indicating an increase in the average size of RuO 2 nanoparticle during the reaction [49] . Consequently, the weakening of the interaction facilitates the volatility and migration of Ru species, leading to the formation of large particles, which in turn reduces the number of active sites and deactivates the catalyst during soot oxidation. These results demonstrate that the single-atom Ru sites anchored on the surface lattice of CeO 2 nanocrystals exhibit high thermal and structural stability during soot oxidation. Nitric oxide (NO) emissions from automobile exhaust are inevitable and can promote the removal efficiency of soot particles through NO oxidation into NO 2 , enhancing soot oxidation via a NO 2 -assisted mechanism [50] . We also investigated the role of NO over single-atom Ru active sites during catalytic soot oxidation (Supplementary Fig. 25a, b ). Interestingly, the catalytic activity of Ru n /CeO 2 catalyst is higher than that of the Ru 1 /CeO 2 catalyst under the sole presence of O 2 . However, with the addition of NO, the T 50 values significantly shift to the lower temperature for both Ru 1 /CeO 2 and Ru n /CeO 2 catalysts. The temperature difference (Δ T 50 ) of Ru 1 /CeO 2 and Ru n /CeO 2 catalysts is 87 and 54 o C under the sole presence of 5 vol% O 2 , and 5 vol% O 2 + 0.2 vol% NO, respectively. This observation indicates that the presence of NO has a more pronounced effect on soot oxidation, emphasizing the critical role of NO activation and oxidation in enhancing catalytic activity for soot oxidation. It suggests that the Ru 1 /CeO 2 catalyst can significantly promote the activation and oxidation of NO, thereby enhancing catalytic activity for soot oxidation via the NO 2 -assistant soot purification mechanism. The catalytic performance for NO oxidation was further evaluated using NO-temperature programmed oxidation (NO-TPO, Fig. 2f ). It is noted that the Ru 1 /CeO 2 catalyst has a higher NO 2 concentration than the Ru n /CeO 2 catalyst. Moreover, the Ru 1 /CeO 2 (305 o C) catalyst exhibits a lower temperature of NO 2 concentration peak comparison with the Ru n /CeO 2 catalyst (315 o C). Therefore, the single-atom Ru sites anchored on the surface lattice of CeO 2 {111} facets exhibit improved catalytic performance for low-temperature NO oxidation compared with the Ru n /CeO 2 catalyst. The relatively low temperature of NO oxidation over the single-atom Ru catalyst indicates that the Ru 1 /CeO 2 catalyst demonstrates excellent activation and oxidation of NO molecules, contributing to its super-catalytic performance for NO 2 -assistant soot oxidation. Identifying active species and reaction pathways during soot oxidation The performance of the catalysts during deep oxidation strongly depends on the presence of surface-active oxygen species, which are generated from activated O 2 molecules by the low-coordinatively unsaturated cation (CUC) sites. Identifying the active species involved in catalyzing soot oxidation is crucial to understanding the reaction mechanism. We investigated the surface density of CUC sites induced by single-atom Ru species using Raman scattering spectra (Fig. 3a ). The strong vibration peak at ~464 cm −1 corresponds to the first-order F 2g symmetry of CeO 2 nanocrystals. Interestingly, the presence of Ru in the Ru 1 /CeO 2 catalyst causes this peak to shifts down by ~7 cm −1 (Supplementary Fig. 26 ), suggesting that the atomically dispersed Ru species either lowers the symmetry of Ce-O bond on the Ru 1 /CeO 2 catalysts or facilitates the transfer of electrons from Ru species to CeO 2 , affecting the electronic structure of the catalyst [51] , [52] . Additionally, the Raman peak centered at ~598 cm −1 corresponds to the defect-induced ( D ) mode of CeO 2 , and its intensity noticeably increases with the introduction of Ru species [53] . For Ru 1 /CeO 2 and Ru n /CeO 2 catalysts, two exclusive peaks at ~682 and ~975 cm −1 indicate the formation of the Ru-O-Ce bond, further confirming the presence state of Ru n+ species in the catalysts [54] . Moreover, a weak peak at ~323 cm −1 can be attributed to RuO 2 formation in Ru n /CeO 2 catalyst [55] . Furthermore, the peak at ~831 cm −1 is assigned to isolated two-electron surface defect sites on oxidized surfaces of Ce-based oxide [56] . To evaluate the surface density of oxygen vacancies, we examined the area ratio of D peak to F 2g peak (denoted as I D / I F2g ) [57] . The Ru 1 /CeO 2 catalyst exhibits the highest I D /I F2g value (Supplementary Fig. 27 ), indicating that the formation of the Ru-O-Ce bond induces electronic transfer from Ru to Ce 4+ , leading to two Ce 4+ ions replaced by two Ce 3+ ions for creating each oxygen vacancy. As a result, the surface density of CUC sites is increased. Fig. 3: Identifying active species and reaction pathways of the catalysts during catalyzing soot oxidation. a Raman spectrum with an excitation wavelength of 532 nm. b H 2 -TPR profiles. c XPS spectra of O 1 s . d The ratio of oxygen species determined by XPS. e Temperature-dependent in-situ DRIFT spectra and ( f ) corresponding contour projection results of NO oxidation on Ru 1 /CeO 2 catalyst (Catalyst, 10 mg; 5 vol% O 2 and 0.2 vol% NO). Full size image The amount of active oxygen species generated by CUC sites can be evaluated using temperature-programmed reduction with H 2 (H 2 -TPR). CeO 2 -M catalyst exhibits a lower reduction temperature (457 and 781 o C) and higher H 2 consumption (1.389 mmol g -1 ) compared to CeO 2 -C catalyst (Fig. 3b and Supplementary Fig. 28 ), indicating that the exposed CeO 2 {111} facets enhance the oxidation property of surface oxygen species. In the H 2 -TPR profile of the Ru n /CeO 2 catalyst, the first peak located at 127 o C is assigned to the reduction of RuO x . However, the reduction of Ru species in the Ru 1 /CeO 2 catalyst occurs at a higher temperature, 173 o C, indicating a stronger interaction between Ru species and the support compared to that in the Ru n /CeO 2 catalyst [56] . The reduction temperature of Ru species in the Ru 1 /CeO 2 catalyst is higher than in the Ru n /CeO 2 , indicating two different existing states of Ru species. The initial H 2 consumption rate reflects the activity of low-temperature surface oxygen species, and for supported Ru catalysts, their values increase more than thirteen-fold compared to bare CeO 2 -M (Supplementary Fig. 29 ), which results in the relatively low ignition temperature ( T 10 ) during catalytic soot oxidation (Supplementary Fig. 13 ). XPS was used to investigate the surface element state in the catalysts. The O 1 s XPS can be deconvoluted into three peaks (Fig. 3c ). Surface peroxy-(O 2 2- ) and super-oxygen (O 2 - ) species, activated by CUC sites, are considered active oxygen species rather than lattice oxygen (O 2- ) during deep oxidation reactions. The percentage of active oxygen species in the single-atom Ru catalyst is the highest (37%) (Fig. 3d ), suggesting that the CUC sites induced by Ru species greatly enhance the adsorption-activation of O 2 molecules, leading to the formation of active oxygen species. This finding is consistent with the analysis result of Ce 3 d XPS which shows that the Ru 1 /CeO 2 catalyst has the highest percent (27.6%) of coordinatively unsaturated Ce 3+ species, resulting from the strong Ru-O-Ce electronic interaction (Supplementary Fig. 30 and Supplementary Table 5 ). This electronic interaction is crucial for boosting the catalytic activity of soot oxidation [56] . The transformation pathways of surface-active species over the catalysts were studied using in-situ DRIFTS. At 50 o C, a series of NO x -containing species is observed on surface of the Ru 1 /CeO 2 catalyst after introduction of NO and O 2 into the reactor (Fig. 3e ). These species include N 2 O 4 dimer (1766 cm -1 ), bridging nitrates (1627 cm −1 ), monodentate nitrites (1422 and 1360 cm -1 ), ionic nitrites (1390 cm -1 ) and nitrates (836 cm -1 ) (Supplementary Table 6 ). As the reaction temperature increases, the three characteristic peaks of ionic nitrites and monodentate nitrites gradually merge into one new peak (1372 cm -1 ), and its intensity increases significantly. At the same time, the peak of bridged nitrates gradually weakens and eventually disappears, while new peaks of anionic (1134 cm −1 ) and bidentate (1043 and 965 cm -1 ) nitrates appear (Fig. 3f ). These changes suggest that the adsorbed NO x species gradually transform into labile NO 3 - intermediates, which subsequently decompose into NO 2 . The Ru n /CeO 2 catalyst exhibits similar evolution processes of in-situ DRIFTS spectra for NO oxidation (Supplementary Fig. 31 ), and the Ru 1 /CeO 2 catalyst exhibits the largest relative intensity of surface NO 3 - at 200 o C (Supplementary Fig. 32 ), indicating that single atomic Ru species significantly promote the transfer from surface active oxygen to NO 3 - intermediate. Finally, the gaseous NO 2 produced by surface nitrate decomposition boosts catalyzing soot oxidation in the NO 2 -assisted mechanism. The electron and energy evolution processes of surface-active intermediate over the catalysts were further investigated through DFT calculations in the following discussion. Insight into the mechanism of single atomic Ru catalyst for soot oxidation To gain insight into NO 2 -assisted catalytic mechanism for soot oxidation over Ru catalysts, the reaction pathways were investigated by DFT calculations. Model active sites of single atom Ru 1 and Ru 10 SNPs were constructed on the surface of CeO 2 (110) facets (Supplementary Fig. 33a-c ). The charge density difference maps of Ru 1 /CeO 2 and Ru 10 /CeO 2 were used to investigate the strong interaction between Ru and CeO 2 , and the extra number of transferred electrons was calculated using Bader charge analyses. The results showed that the Ru 1 model can donate 1.46 e - to CeO 2 support (Supplementary Fig. 34a-c ), while Ru 10 model transfers a total of 1.26 e - , indicating a stronger electronic interaction between Ru 1 and CeO 2 , which boosts the formation of CUC sites compared to Ru 10 SNPs (Supplementary Fig. 35a-c ). The reaction pathways and relative energy ( E ) during catalyzing NO oxidation can be divided into six stages as follows (Fig. 4 ): first, a gaseous O 2 molecule adsorbs on the unsaturated coordination Ce site (Ce-O-Ru) over the catalyst surface through O-O-Ce bond to form surface adsorption O 2 * (IM1). The adsorption energy of O 2 ( E ads (O 2 )) is -0.9 and -0.53 eV for Ru 1 /CeO 2 and Ru 10 /CeO 2 , respectively, indicating that the single Ru site easily adsorbs O 2 molecule. The calculated charge density difference shows that the O 2 molecule can be adsorbed on coordination unsaturated Ce atom of Ru 1 /CeO 2 and Ru 10 /CeO 2 , with a total net charge transfer from Ru 1 /CeO 2 surface to O 2 being 0.56 e - (Supplementary Fig. 36a, b ) and 0.44 e - for Ru n /CeO 2 catalyst (Supplementary Fig. 37a, b ). The adsorbed O 2 molecule over Ru 1 /CeO 2 catalyst gains the more electrons, facilitating the activation of O = O bond. Second, one NO molecule adsorbs on the Ru site of the catalyst surface through the O-N-Ru bond to form surface NO species (IM2). The NO adsorption energy ( E ads (NO)) of Ru 10 /CeO 2 (-2.82 eV) is lower than that of Ru 1 /CeO 2 (-1.63 eV), and this strong adsorption capacity is not conducive to the subsequent reaction over Ru 10 /CeO 2 . Third, the O-O bond of the adsorbed O 2 is activated to dissociate into atomic O* species, and adsorbed NO combines with O* to form the surface intermediate NO 2 * species (IM3). The reaction barriers for these steps are 0.9 and 1.23 eV with the corresponding transition states (TS1) of Ru 1 /CeO 2 and Ru 10 /CeO 2 , respectively. Fourth, the NO 2 species desorb from the catalyst surface (IM4). The NO 2 desorption energy ( E des (NO 2 )) for Ru 1 /CeO 2 (1.01 eV) is lower than that of Ru 10 /CeO 2 (2.60 eV), indicating that the desorption of NO 2 molecules over the single atomic Ru site is easier than that of Ru 10 site. This result in the rapid formation of NO 2 on the surface of Ru 1 /CeO 2 catalyst, a crucial step during soot oxidation. Fifthly, an additional NO molecule adsorbs on the O* to form ONO* (IM5). Finally, the formation of NO 2 * species desorbs from the catalyst surface, completing the reaction cycle (FS). The NO 2 desorption energy ( E des (NO 2 )) for Ru 1 /CeO 2 (1.70 eV) is lower than that of Ru 10 /CeO 2 (2.15 eV), indicating that the NO 2 molecule was easily desorbed from the catalyst surface. Based on the above results, we found that NO molecules prefer to adsorb on Ru active sites on the surface of the catalysts, while O 2 molecules are strongly adsorbed on the CUC sites. The rate-determining step of NO oxidation at the Ru-CeO 2 interface is the formation of NO 2 * intermediate species. The stronger oxidizing NO 2 can migrate to the soot surface along with the reaction gas flow and oxidize them to form CO 2 via the indirect pathway (NO + 1/2O 2 → NO 2 and NO 2 + soot → CO 2 ). These DFT calculation results for NO oxidation are consistent with our experimental findings. The single active Ru site easily boosts NO oxidation to NO 2 intermediate, which is beneficial to further promote soot oxidation. Fig. 4: DFT calculations of Ru 1 /CeO 2 and Ru 10 /CeO 2 catalysts for NO oxidation. Reaction steps during catalyzing NO oxidation (Ru atom, black green; Ce atom, gray; O atom, red; N atom, blue). Color code: Ru 1 /CeO 2 (brown line) and Ru 10 /CeO 2 (blue line). Full size image We successfully fabricated stabilizing single-atom Ru sites on the surface lattice of nanoflower-like CeO 2 . The Ru 1 O 5 coordination structure in the Ru 1 /CeO 2 catalyst demonstrated remarkable thermal stability and activity in boosting the adsorption and activation of NO and O 2 molecules, resulting in the formation of the crucial NO 2 intermediate, which plays a key role in the NO 2 -assisted catalytic mechanism for soot oxidation. Therefore, the Ru 1 /CeO 2 catalyst exhibits excellent intrinsic catalytic performance with a high turnover frequency (TOF Ru =0.218 h −1 ) and low apparent activation energy ( E a = 75.2 kJ mol -1 ) during auto-exhaust soot oxidation, surpassing both Ru nanoparticle (TOF Ru =0.023 h -1 ) and commercial Pt-based catalysts. Moreover, the single-atom Ru 1 /CeO 2 catalyst demonstrates exceptional selectivity of the CO 2 product (>99%) and remarkable durability during catalytic soot oxidation. This high-efficiency of the single-atom Ru catalyst offers a promising avenue for designing a considerably low-cost auto-exhaust treatment system, moving away from the reliance on costly Pt and Pd-based catalysts. The findings are also of significant importance for the further development of single-atom catalysts in the areas of deep oxidation and activated O 2 reactions. The single-atom Ru catalyst paves the way for environmentally friendly and efficient exhaust treatment technologies, contributing to cleaner air and sustainable development. Chemicals Cerium (III) nitrate hexahydrate, acrylamide, and glucose were purchased from Aladdin Technology Co., Ltd. Standard ammonia solution (25 wt%) was purchased from Macklin Technology Co., Ltd. Ruthenium (III) chloride hydrate was purchased from J&K Scientific Ltd. Ethanol was purchased from Sigma Aldrich. All reagents and solvents were of analytical grade and used as received without additional purification. Catalysts preparation Syntheses of nanoflower-like CeO 2 microspheres and prepared conventional CeO 2 nanoparticles the nanoflower-like CeO 2 microsphere was synthesized by the hydrothermal method [58] . The glucose (1.98 g, 0.010 mol) was dissolved into 80 mL of deionized water, and the addition of acrylamide (1.05 g, 0.015 mol) and hydrated cerium (III) nitrate (2.17 g, 0.005 mol) was stirred to form a transparent solution. Then, the standard ammonia solution (3.2 mL, 25 wt%) was dropwise to the above solution, and the solution became the sol with vigorous stirring at room temperature for 5 h. The color of the gelatinous mixture turned dark brown at the pH value of 10. Subsequently, the mixture was transferred into a 100 mL Teflon-lined autoclave and kept at 180 o C for 72 h. After the natural cooling of the autoclave to room temperature, the sediment was separated by centrifugation, and the sample was washed with deionized water and ethanol three times. The nanoflower-like CeOHCO 3 microsphere was obtained by drying at 80 o C for 12 h, and was further two-steps calcined at 600 o C for 4 h in N 2 and at 500 o C for 4 h in air. Finally, nanoflower-like CeO 2 microsphere (denoted as CeO 2 -M) was obtained. Conventional CeO 2 nanoparticles (CeO 2 -C) as reference sample was synthesized by the deposition-precipitation method. Cerium (III) nitrate hexahydrate (0.50 g) was dissolved into 20 mL of deionized water. Then, a standard ammonia solution (5 mL) was added dropwise under vigorous stirring. After aging for 30 min, the obtained product was washed with deionized water and ethanol. The product was dried at 80 o C for 12 h and calcined at 500 o C for 4 h in an air atmosphere to obtain general CeO 2 -C. Syntheses of nanoflower-like Ru 1 /CeO 2 and Ru n /CeO 2 catalysts The nanoflower-like CeO 2 -supported single-atom Ru (Ru 1 /CeO 2 ) catalyst was synthesized by a gas bubbling-assisted membrane deposition (GBMD) method [33] . CeO 2 -M support (50 mg) was dispersed into deionized water (400 mL) with vigorous stirring, and 0.646 mL RuCl 3 ·3H 2 O solution (0.01 g mL −1 ) was dropwise added into the above light-yellow slurry (denoted as Beaker I). A stabilizer (polyvinyl pyrrolidone, the molar ratio of Ru/PVP unit is 1/100) was then transferred to Beaker I. A peristaltic pump with a rotation speed of 200 rpm was developed to form tubal cycling of the above solution mixture between the membrane reactor and Beaker I at a flow rate of 400 mL min −1 . In the membrane reactor, the solution mixture flowed in the glass tube and outside the ceramic tubes. Prepared ammonia solution (1 mL standard ammonia solution was added to 40 mL deionized water) as a precipitant was immitted into the membrane reactor by a constant flow pump at a flow rate of 0.2 mL min −1 . The ammonia solution infiltrated through the abundant holes on the walls of the two ceramic tubes into the glass tube, and the deposition of Ru ions occurred immediately until all the ammonia solution was completely consumed. The color of the slurry changed from light brown to dark gray, indicating that the Ru species were deposited. The mixture was filtered and washed with deionized water and ethanol three times, and the product was dried at 60 o C for 12 h. Finally, the sample was calcined to obtain a single-atom Ru catalyst at 500 o C for 4 h in air, denoted as Ru 1 /CeO 2 . The CeO 2 -M supported Ru nanoparticle (Ru n /CeO 2 ) catalyst was prepared by using the gas bubbling-assisted membrane reduction method. This process is similar to GBMD, except that the high stoichiometric regents of RuCl 3 ·3H 2 O (0.01 g mL −1 , 5.167 mL) and PVP (Ru/PVP unit is 1/100). Moreover, NaBH 4 solution as a reductant (the molar ratio of NaBH 4 /Ru is 5/1) was immitted into the membrane reactor by a constant flow pump at a flow rate of 0.2 mL min −1 . The NaBH 4 solution (40 mL) infiltrated through the abundant holes on the walls of the two ceramic tubes into the glass tube, and the reduction of Ru ions occurred immediately until all the NaBH 4 solution was completely consumed. The mixture was filtered and washed with deionized water and ethanol three times, and the product was dried at 60 o C for 12 h. Finally, the sample was calcined at 500 o C for 4 h in air, denoted as Ru n /CeO 2 . Characterizations Powder X-ray (XRD) patterns were obtained by a diffractometer (Bruker D8 advance) using Cu-Kα radiation to obtain the phase structure of all as-prepared catalysts. The Ru K-edge X-ray absorption near edge structure (XANES) and extended X-ray absorption fine structure (EXAFS) experiments were carried out on the experiment assist system of SSRF and beamline BL13SSW and BL06B of the Shanghai Synchrotron Radiation Facility (SSRF). Raman spectra of all catalysts were measured on an inVia Reflex-Renishaw spectrometer with an excitation wavelength of 532 nm. Scanning electron microscopy (SEM), transmission electron microscope (TEM) and high-resolution transmission electron microscope (HRTEM) images were obtained by ZEISS Gemini SEM 300 and JEOL JEM LaB 6 2100, respectively. STEM-ADF images and EDX mapping were obtained by Hitachi HF5000, working at an accelerating voltage of 200 kV. The actual loading amounts of Ru in catalysts were determined by ICP-OES (Perkin Elmer, OPTIMA 7300 V). The pore size and specific surface area of catalysts were characterized by nitrogen adsorption−desorption experiments (Micromeritics TriStar-II 3020). Temperature-programmed reduction with H 2 (H 2 -TPR) was carried out on a fixed-bed device. The surface element valence state was detected by X-ray photoelectron spectra (XPS, XPSPHI−1600 ESCA spectrometer). NO-TPO experiments were carried out on a fixed-bed tubular quartz reactor with flowed the gaseous contained O 2 (5 vol%) and NO (0.2 vol%) balanced with N 2 (50 mL min −1 ), and the products can be detected by online FT-IR. In situ diffuse infrared Fourier transforms spectra (in-situ DRIFTS) were carried on a Bruker FT-IR spectrometer (TENSOR II) equipped with a liquid nitrogen-cooling mercury-cadmium-telluride (MCT) detector. Before the in-situ CO-DRIFTS adsorption and desorption experiment, the sample (10 mg) was loaded into high-temperature IR cell with a ZnSe window (Pike Technologies), and pretreated in a 10 vol% H 2 and balanced with N 2 flow rate of 30 mL min −1 at 300 o C for 30 min. After cooling down to 50 o C under N 2 flow (30 mL min −1 ) for 10 min, the background was collected. For the CO adsorption step, the CO (10 vol% CO in N 2 balance) gas was fed into the cell at a flow rate of 30 mL min −1 for 30 min up to adsorption saturation. For the CO desorption, N 2 flow (30 mL min −1 ) was purged into the cell to remove adsorbed CO, and the spectra were recorded at an apart of 2 min. In-situ DRIFTS of NO oxidation test, the catalyst (10 mg) was added into high-temperature IR cell with ZnSe window, and heated in N 2 flow at 200 o C for 30 min to remove adsorbed H 2 O and other materials. After cooling down to 50 o C with N 2 atmosphere, the background spectrum was recorded. Finally, the O 2 (5 vol%), NO (0.2 vol%) and balanced with N 2 were fed into cell at a flow rate of 50 mL min −1 . IR spectra of the catalysts were recorded in a flow of 0.2 vol% NO/5 vol% O 2 /N 2 balance (50 mL min −1 ) under heating from 50 to 400 o C. Catalytic activity and kinetic tests The catalytic activity for soot oxidation was evaluated by soot-TPO in a tubular quartz reactor using Printex-U as model soot particles. The loose contact was obtained by mixing the catalyst (100 mg) and soot (10 mg) with a spoon for 10 min, and the tight contact was obtained by grinding the above mixture for 10 min. The reaction temperature in soot-TPO rises from 150 to 550 o C with a rising rate of 2 o C min −1 . The reaction gases were composed of 5 vol% O 2 and 0.2 vol% NO balanced with Ar, and the total flow rate was 50 mL min −1 passed through the mixture. The gas product of CO 2 and CO in the outlet gas was monitored by an online gas chromatograph (GC 9890B, Shanghai). The catalytic performance was evaluated by the TOF Ru , which can be defined by the ratio of the isothermal reaction rate ( R ) to the actual amount of Ru-supported in the catalysts. The temperature at 10%, 50%, and 90% of soot conversion from soot-TPO test denotes T 10 , T 50 , and T 90 , respectively. The selectivity of CO 2 ( S CO2 ) can be calculated by the ratio of CO 2 concentration to the sum of CO and CO 2 concentration, and the S CO2 was calculated by the following formula: 
    S_CO2(%)=[CO_2]_out/[CO]_out+[CO_2]_out
 (1) Here, the [CO 2 ] out and [CO] out represent the outlet CO 2 and CO concentration (ppm), respectively. S CO2 m was defined as S CO2 with the maximum value of CO 2 concentration. The R values can be obtained by isothermal reaction at 280 o C for soot oxidation, the conversion of soot remains basically unchanged and the conversion rate is less than 10%. The R values for all catalysts were calculated by the slopes of the soot conversion amount with time, which are reflected in the concentration of CO 2 per unit of time. The soot conversion rate ( R ) was calculated as following [59] : 
    R(molg^-1min^-1)=QC/22400×m
 (2) Where Q represents the gas flow rate (mL min −1 ), C represents the concentration of CO 2 measured by isothermal reactions (ppm), and m represents the weight of the catalyst (g). The active oxygen ( O a ) amount can be obtained by isothermal anaerobic titrations [31] . The TOF Ru value of the Ru/CeO 2 catalyst can be calculated by the following equation: 
    TOF_Ru(h^-1)=(R2-R1)M× 6×10^-6/mw
 (3) Here, the R2 and R1 represent the isothermal reaction rate for Ru/CeO 2 and CeO 2 catalysts (μmol g −1 min −1 ), respectively. M is the atomic weight of Ru (101.07 g mol −1 ), m is the mass of the catalyst (g) and the w (wt.%) is the actual loading amount of Ru species on the surface of CeO 2 . The apparent activation energy ( E a ) can be calculated by the Coats-Redfern interregnal method [60] . The E a values are obtained by the following equation: 
    ln[-ln(1-α)/T^2]= ln[AR/βEa(1-2RT/Ea)]-Ea/RT
 (4) Here, the α is the conversion value of soot, %. T is the reaction temperature, K. A is the pre-exponential factor, s −1 . E a is the apparent activation energy, kJ mol −1 . R represents the ideal gas constant, 8.314 J mol −1 K −1 . β represents the heating rate, K min −1 . The stability of catalysts was evaluated by Time-TOF Ru and recycling soot-TPO tests. For the Time-TOF Ru test, a spatula was used to mix soot (20 mg) and catalyst (200 mg) thoroughly to form loose contact. The mixture was heated on a fixed-bed tubular quartz microreactor with an inner diameter of 6 mm, and heated from 50 to 280 o C at a heating rate of 2 o C min −1 under a reactant gas flow (50 mL min −1 ) of O 2 (5 vol%) and NO (0.2 vol%) balanced with Ar. The reaction temperature was kept at 280 o C (lasting for 400 min) in an approximate kinetic regime because the conversion of soot oxidation was low (10%) and nearly constant over time. The outlet gas concentration of CO and CO 2 is detected by an online gas chromatograph. When the temperature reaches 280 o C, the outlet gas concentration is detected for the first time as the starting point. Based on the above process, the production CO 2 concentration of Ru/CeO 2 and CeO 2 catalysts can be obtained at specific times, respectively. The CO 2 produced by the bare Ru species can be defined as the concentration produced by Ru/CeO 2 subtraction of the concentration of CO 2 produced by the CeO 2 . The TOF Ru value was calculated as follows: 
    TOF_Ru(h^-1)=C_CO2^pQM× 6×10^-5/22400×mw
 (5) Where the \({{{{{{\rm{C}}}}}}}_{CO2}^{p}\) represents the produced CO 2 concentration (ppm) by the bare Ru species, the value can be defined as the concentration produced by Ru/CeO 2 subtraction of the concentration of CO 2 produced by the support CeO 2 . Q represents the gas flow rate (mL min −1 ), M is the atomic weight of Ru (101.07 g mol −1 ), m is the mass of the catalyst (g) and the w (wt.%) is the actual loading amount of Ru species on the surface of CeO 2 . Finally, the profile of Time-TOF Ru and the selectivity of CO 2 over Ru 1 /CeO 2 and Ru n /CeO 2 catalysts were gained within 400 min. For the cyclic stability test, the catalyst was recycled after the first test of soot-TPO. The detailed process is as follows: firstly, the catalyst was taken out from the reaction quartz tube and then the quartz cotton was cleaned off from the surface of the catalyst (this process loses about 2% of the catalyst mass). Each time, the used catalyst was mixed with 10 mg soot particles, and the next activity test (soot-TPO) was performed, the values of T 10 , T 50 , T 90 and S CO2 m for Ru/CeO 2 catalysts can be obtained. The above experimental process was repeated six times, and six groups of activity data were finally acquired, while no additional catalyst was added for each test during six cycles of soot-TPO. Density functional theory (DFT) calculations DFT calculations were carried out by using the VASP package code [61] . The exchange-correlation energy function was described in the Pardew-Burke-Ernzerhof (PBE) generalized gradient approximation (GGA) [62] . The kinetic cutoff energy is 400 eV for the plane-wave basis set, and the k point was set to the γ point in the Brillouin zone. All calculations for CeO 2 models were performed by the DFT + U method for the present study. The value of U eff was set to 5 eV for Ce 4 f electrons. CeO 2 supercells (2 x 4) were built, with (110) surfaces exposed. The bottom two atomic layers were fixed during all calculations. The thinness of the vacuum layer for all the models was set as 15 Å. Combined with the results of STEM-ADF and EXAFS characterizations, one of the Ce atoms in the surface layer was replaced by a Ru atom to simulate the single-atom Ru structure, and the Ru nanoparticles contain 10 atoms in the Ru n /CeO 2 model [63] . The adsorption and desorption energy were calculated by the equation: 
    E_ads=E_MS-E_S-E_M
 (6) 
    E_des=E_S+E_M-E_MS
 (7) Where E ads is the adsorption energy, E des is the desorption energy, E MS is the total energy of a surface slab with the adsorbate, and E S is the energy of pure substrate. E M represents the energy of an adsorbate molecule. The climbing image-nudged elastic band (CI-NEB) code was used to identify the reaction coordinates from IS to FS [64] , [65] , which located the transition state (TS). The activation energy ( E a) and reaction energy ( E r ) were determined with the following equation: 
    E_a=E_TS-E_FS
 (8) 
    E_r=E_FS-E_IS
 (9) Where E IS , E TS , and E FS represent the energy of IS, TS, and FS, respectively.